Distinct pathways mediate axon degeneration during apoptosis and axon-specific pruning Neurons can activate pathways that destroy the whole cell via apoptosis or selectively degenerate only the axon (pruning). Both apoptosis and axon degeneration require Bax and caspases. Here we demonstrate that despite this overlap, the pathways mediating axon degeneration during apoptosis versus axon pruning are distinct. While Caspase-6 is activated in axons following nerve growth factor deprivation, microfluidic chamber experiments reveal that Caspase-6 deficiency only protects axons during axon-specific but not whole-cell (apoptotic) nerve growth factor deprivation. Strikingly, axon-selective degeneration requires the apoptotic proteins Caspase-9 and Caspase-3 but, in contrast to apoptosis, not apoptotic protease activating factor-1. Additionally, cell bodies of degenerating axons are protected from caspase activation by proteasome activity and X-linked inhibitor of apoptosis protein. Also, mature neurons restrict apoptosis but remain permissive for axon degeneration, further demonstrating the independent regulation of these two pathways. These results reveal insight into how neurons allow for precise control over apoptosis and axon-selective degeneration pathways, thereby permitting long-term plasticity without risking neurodegeneration. Neurons execute one of two critical self-destruct programs to properly shape the developing nervous system: apoptosis, which destroys the entire neuron, and axon degeneration, which removes unnecessary axon branches to refine neuronal connections [1] , [2] . While extensive neuronal apoptosis occurs during development [3] , the apoptotic pathway becomes highly restricted once neurons are integrated into the nervous system, enabling neurons to survive for the lifetime of the organism [4] , [5] , [6] , [7] . In contrast, the selective pruning of axons is critical not only for establishing specific neuronal circuitry during development but also for permitting plasticity in the adult nervous system [8] , [9] , [10] . Although axons are destroyed during both apoptosis and axon-specific degeneration, whether exactly the same pathway mediates axonal destruction in these two contexts has not been specifically examined. The key mediators of the apoptosis pathway are caspases, a family of cysteine proteases that cleave specific cellular substrates to cause rapid cell death [11] . Apoptotic signalling cascades converge on and activate Bax, a proapoptotic member of the Bcl-2 family, resulting in the release of cytochrome c (cyt c ) from the mitochondria. Released cyt c binds to Apaf-1 (apoptotic protease activating factor-1), which recruits procaspase-9 to form the apoptosome complex. Autoactivation of caspase-9 (Casp9) leads to the cleavage and activation of caspase-3 (Casp3), resulting in cell death. Caspase activation in neurons is strictly regulated by XIAP (X-linked inhibitor of apoptosis protein), which binds to and inhibits cleaved Casp9 and Casp3. Thus, inactivation of XIAP is necessary for caspase-mediated apoptosis in neurons [12] . Any overlap between neuronal apoptosis and axon-specific degeneration was initially dismissed due to the lack of active Casp3 detection in degenerating axons and the inability of Casp3-specific inhibition to protect axons [13] , [14] , [15] . Interestingly, however, recent studies point to significant overlap between these two pathways. For example, the Bcl-2 family proteins have been shown to modulate axon degeneration as deficiency of Bax or overexpression of anti-apoptotic protein Bcl-XL both protect axons following axon-specific nerve growth factor (NGF) deprivation [13] , [16] , [17] . Furthermore, several caspases—specifically Casp9, Casp3 and caspase-6 (Casp6)—have now all been implicated in axon degeneration [13] , [17] , [18] , [19] , [20] , [21] , [22] , [23] . These results raise several interesting points. If the effectors of apoptosis and axon degeneration are identical, how do neurons activate axon-selective degeneration without triggering apoptosis? Alternatively, are there key differences that remain unidentified that allow neurons to precisely activate one but not the other pathway? In this study, we examine the molecular intersection between axon degeneration and apoptosis. We report that the pathways mediating axon degeneration in the context of apoptosis versus localized, axon-specific degeneration are distinct. We also find that activities of the proteasome and XIAP are important for restricting caspase activation to the axons during axon-selective degeneration. Importantly, we show that mature neurons, which restrict apoptosis, are still capable of undergoing axon-specific degeneration, further supporting our conclusion that neuronal apoptosis and axon degeneration are mediated by different mechanisms. The distinct regulation of these two pathways is essential for maintaining life-long neuronal plasticity without risking neurodegeneration. Axon-selective pruning requires Casp6 As Casp6 has emerged as an important mediator of axon degeneration, we examined whether Casp6 is activated in multiple models of axon degeneration. We subjected whole cultures of primary mouse sympathetic neurons to various insults in vitro , including NGF deprivation, DNA damage with etoposide, endoplasmic reticulum stress with tunicamycin and microtubule destabilization with vinblastine. Consistent with recent reports [17] , despite the ability of all treatments to induce extensive axon degeneration ( Fig. 1a ), we detected robust axonal Casp6 staining selectively following NGF deprivation but not other insults ( Fig. 1b ). NGF deprivation is known to induce apoptosis in neurons resulting in both soma and axon degeneration. To test whether Casp6 was required for axon degeneration in this model, we isolated neurons from wild-type and Casp6-deficient mice and deprived them of NGF. Surprisingly, Casp6 deficiency did not prevent axon degeneration in NGF-deprived neurons; Casp6-deficient neurons underwent apoptosis and exhibited soma and axon degeneration just as seen with wild-type neurons ( Fig. 2a ). 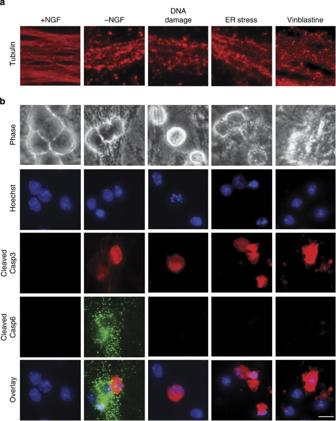Figure 1: Casp6 activation in axons is selective to NGF deprivation. (a) Wild-type (WT) sympathetic neurons (5 DIV) were treated with the following conditions to induce axon degeneration, respectively: NGF deprivation (-NGF), 20 μM etoposide (DNA Damage), 2.5 μM tunicamycin (endoplasmic reticulum (ER) Stress) and 1 μM vinblastine (to induce microtubule destabilization). NGF-maintained neurons served as controls. Neurons were fixed and immunostained for tubulin upon axon beading and fragmentation. (b) Neurons were treated as described inaand immunostained for cleaved Casp3 and cleaved Casp6. Nuclei were labelled with Hoechst. Scale bar, 20 μm. Figure 1: Casp6 activation in axons is selective to NGF deprivation. ( a ) Wild-type (WT) sympathetic neurons (5 DIV) were treated with the following conditions to induce axon degeneration, respectively: NGF deprivation (-NGF), 20 μM etoposide (DNA Damage), 2.5 μM tunicamycin (endoplasmic reticulum (ER) Stress) and 1 μM vinblastine (to induce microtubule destabilization). NGF-maintained neurons served as controls. Neurons were fixed and immunostained for tubulin upon axon beading and fragmentation. ( b ) Neurons were treated as described in a and immunostained for cleaved Casp3 and cleaved Casp6. Nuclei were labelled with Hoechst. Scale bar, 20 μm. 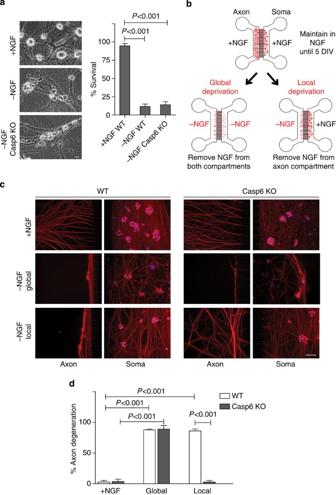Figure 2: Casp6 is required for axon degeneration during axon pruning but not apoptosis. (a) Wild-type (WT) and Casp6-deficient (Casp6 KO) neurons (5 DIV) were NGF-deprived for 24 h. WT neurons maintained in NGF served as a control. Scale bar, 10 μm. (b) Microfluidic chamber model of global deprivation, which induces soma and axon degeneration and local deprivation, which results in axon-selective degeneration. (c) WT and Casp6-deficient neurons were NGF maintained, globally deprived or locally deprived. Neurons were immunostained for tubulin and nuclei were labelled with Hoechst. Scale bar, 50 μm. (d) Quantification of axon degeneration for conditions shown inc. Data represent the mean±s.e.m. (n=3).P-values were calculated using an unpairedt-test. Full size image Figure 2: Casp6 is required for axon degeneration during axon pruning but not apoptosis. ( a ) Wild-type (WT) and Casp6-deficient (Casp6 KO) neurons (5 DIV) were NGF-deprived for 24 h. WT neurons maintained in NGF served as a control. Scale bar, 10 μm. ( b ) Microfluidic chamber model of global deprivation, which induces soma and axon degeneration and local deprivation, which results in axon-selective degeneration. ( c ) WT and Casp6-deficient neurons were NGF maintained, globally deprived or locally deprived. Neurons were immunostained for tubulin and nuclei were labelled with Hoechst. Scale bar, 50 μm. ( d ) Quantification of axon degeneration for conditions shown in c . Data represent the mean±s.e.m. ( n =3). P -values were calculated using an unpaired t -test. Full size image These results were unexpected because recent studies have shown that Casp6 is required for axon degeneration [13] , [20] . However, in these studies, neurons were cultured in compartmentalized chambers and NGF was withdrawn from only the axons. Thus, we examined whether neurons activate a Casp6-dependent or -independent pathway to degenerate axons based on the spatial localization of NGF deprivation signal. We generated microfluidic chambers that permit the physical separation and fluidic isolation of soma and distal axons [24] . The microfluidic chambers allow local NGF withdrawal from distal axons in the axon compartment while maintaining NGF on the cell bodies and proximal axons in the soma compartment ( Fig. 2b ). This axon-specific NGF withdrawal, termed local deprivation, results in axon-specific degeneration in wild-type neurons within 24–48 h. Alternatively, we can also withdraw NGF from both compartments, termed global deprivation, to induce whole-cell degeneration via apoptosis. Using microfluidic chambers to clearly distinguish axon degeneration caused by apoptosis versus that during axon-specific NGF deprivation, we subjected wild-type and Casp6-deficient neurons to global and local deprivation. Our results show that while Casp6 deficiency is indeed able to block axon degeneration with local deprivation, it is incapable of doing so with global deprivation ( Fig. 2c ; Supplementary Fig. S1 ). These results indicate that the Casp6-mediated pathway of axon degeneration induced during local deprivation is distinct from the pathway utilized by dying neurons to degenerate their axons. Thus, neurons appear to have Casp6-dependent and Casp6-independent pathways to degenerate their axons, and the specific location of NGF withdrawal (axon versus whole cell) determines which pathway becomes activated. Apaf-1-independent axon pruning requires Casp9 and Casp3 The requirement of Casp6 in the axon-selective degeneration pathway but not apoptosis indicates that these two pathways are distinct. However, deficiency of Bax protects against both neuronal apoptosis and local deprivation-induced axon degeneration [13] , [16] . Thus, the apoptotic pathway intersects with the axon degeneration pathway. As death receptor 6 (DR6) has been implicated in Casp6 activation in axon degeneration [13] , we first examined whether the death receptor (DR) apoptotic pathway, also known as the extrinsic pathway, was important for axon degeneration. In the extrinsic pathway, activation of caspase-8 can either directly activate Casp3 or cleave Bid, a proapoptotic member of the Bcl-2 family of proteins, which then activates Bax [25] . However, neither Bid-deficiency nor caspase-8-specific inhibition blocked axon degeneration during local deprivation ( Supplementary Fig. S2a,b ). We next tested whether components of the mitochondrial apoptotic pathway are critical for axon-selective degeneration using mice deficient in the key components of this pathway. As anticipated, Bax-deficient axons were protected during local deprivation and lacked Casp6 activation ( Fig. 3a–c ). Both Casp9 and Casp3 were also required for axon degeneration following local deprivation as axons deficient for these respective caspases were protected ( Fig. 3a–c ). Indeed, we detected active Casp3 in locally deprived wild-type axons, indicating that Casp3 is activated during axon-selective degeneration ( Fig. 3b ). Interestingly, we also examined the status of cleaved Casp6 in these knockout neurons that were locally deprived of NGF. While no active Casp6 staining was detected in locally deprived Bax- or Casp9-deficient neurons, we observed positive staining in the Casp3-deficient neurons, albeit to a reduced extent than seen in wild-type neurons ( Fig. 3a ). These results suggest that Casp6 cleavage occurs downstream of Bax and Casp9. Importantly, Casp3 appears to be required for full Casp6 activation in locally deprived axons. 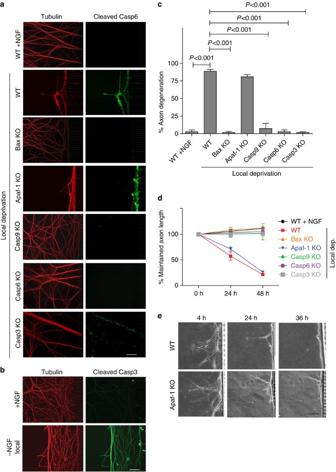Figure 3: Axon-selective degeneration is Apaf-1-independent but requires Casp9 and Casp3. (a) Sympathetic neurons (5 DIV) from mice deficient for Bax, Apaf-1, Casp9, Casp6 and Casp3 were locally deprived in microfluidic chambers. NGF-maintained and locally deprived wild-type (WT) littermate neurons served as controls. Neurons were immunostained for tubulin and cleaved Casp6. (b) WT neurons were locally deprived for 24 h and probed for cleaved Casp3. NGF-maintained neurons served as controls. (c) Quantification of axon degeneration for conditions shown ina. (d) Quantification of maintained axon length over time during local deprivation for all conditions shown ina. All data represent the mean±s.e.m. (n=3). (e) Phase images of the same axons over a 36-h time course of local deprivation demonstrate similar degeneration kinetics between WT and Apaf-1-deficient axons. AllP-values were calculated using an unpairedt-test. Scale bars, 50 μm. Figure 3: Axon-selective degeneration is Apaf-1-independent but requires Casp9 and Casp3. ( a ) Sympathetic neurons (5 DIV) from mice deficient for Bax, Apaf-1, Casp9, Casp6 and Casp3 were locally deprived in microfluidic chambers. NGF-maintained and locally deprived wild-type (WT) littermate neurons served as controls. Neurons were immunostained for tubulin and cleaved Casp6. ( b ) WT neurons were locally deprived for 24 h and probed for cleaved Casp3. NGF-maintained neurons served as controls. ( c ) Quantification of axon degeneration for conditions shown in a . ( d ) Quantification of maintained axon length over time during local deprivation for all conditions shown in a . All data represent the mean±s.e.m. ( n =3). ( e ) Phase images of the same axons over a 36-h time course of local deprivation demonstrate similar degeneration kinetics between WT and Apaf-1-deficient axons. All P -values were calculated using an unpaired t -test. Scale bars, 50 μm. Full size image Next, we examined the importance of the key apoptotic protein Apaf-1 in axon degeneration. Similar to neurons deficient for Bax, Casp9 and Casp3, neurons deficient for Apaf-1 are protected from apoptosis induced by NGF deprivation [26] . Strikingly, Apaf-1 deficiency did not block axon-selective degeneration following local deprivation ( Fig. 3 ; Supplementary Fig. S2c ). Similar to wild-type neurons, robust Casp6 activation was also seen in Apaf-1-deficient neurons ( Fig. 3a ). These results indicate that while axon-selective degeneration is Casp9- and Casp3-dependent, it is Apaf-1-independent. As active Bax is known to trigger mitochondrial cyt c release during apoptosis, we also examined the status of cyt c in deprived axons. Control axons in the presence of NGF-maintained cyt c in the mitochondria and global deprivation triggered its release (as indicated by the loss of cyt c staining). Our results show that local deprivation also induced the release of cyt c from mitochondria in the axon compartment ( Fig. 4 ). 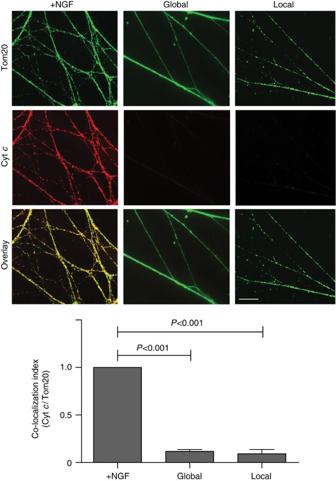Figure 4: Local deprivation triggers cytcrelease in axons. Neurons (5 DIV) were NGF maintained, globally deprived or locally deprived in the presence of pan-caspase inhibitor (25 μM quinolyl-Val-Asp-OPh, or QVD) for 36 h and probed for cytcand the mitochondrial marker Tom20. Quantification of the co-localization index (ImageJ) for cytcand Tom20 is shown below. Data represent the mean±s.e.m. (n=3). Scale bar, 10 μm. AllP-values were calculated using an unpairedt-test. Figure 4: Local deprivation triggers cyt c release in axons. Neurons (5 DIV) were NGF maintained, globally deprived or locally deprived in the presence of pan-caspase inhibitor (25 μM quinolyl-Val-Asp-OPh, or QVD) for 36 h and probed for cyt c and the mitochondrial marker Tom20. Quantification of the co-localization index (ImageJ) for cyt c and Tom20 is shown below. Data represent the mean±s.e.m. ( n =3). Scale bar, 10 μm. All P -values were calculated using an unpaired t -test. Full size image Together, these results show that axon degeneration during apoptosis versus axon-selective pruning have some overlap but also key differences. While both pathways require Bax, Casp9 and Casp3, they diverge at the requirements of Casp6 (required only for axon-selective pruning) and Apaf-1 (required only for axon degeneration during apoptosis). XIAP and the proteasome protect the soma during axon pruning The unexpected involvement of proapoptotic caspases in axon degeneration raises a key question of how neurons can limit caspase activity to axons without increasing the risk of apoptosis at the soma. While some have reported proteasome inhibition to inhibit axon degeneration [27] , [28] others have reported the opposite effect [29] , [30] . Recently, Casp6 activity was reported to be enhanced by proteasome inhibition [31] , [32] . Indeed, we detected Casp6 activation and axon degeneration at an earlier timepoint when proteasome activity was inhibited with Bortezomib ( Fig. 5a ; Supplementary Fig. S3a ) or MG132 (data not shown). Equally striking, proteasome inhibition made the cell bodies of locally deprived axons more permissive for caspase activation; significantly more Casp3- and Casp9-positive cell bodies were observed in locally deprived, proteasome-inhibited chambers than those that had been locally deprived without proteasome inhibitor ( Fig. 5b ). Proteasome inhibition alone did not induce Casp3 activation in NGF-maintained neurons ( Fig. 5a ). Also, the increased axon degeneration seen with proteasome inhibition after local deprivation was Casp3-dependent, indicating that this degeneration was not due to nonspecific toxicity of proteasome inhibition ( Fig. 5d ). 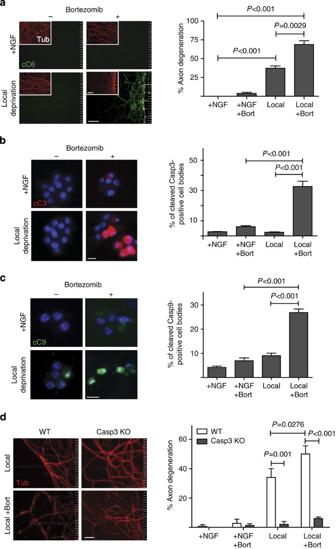Figure 5: The proteasome restricts caspase activation to axons during axon-specific degeneration. (a) Wild-type (WT) neurons were NGF maintained or locally deprived in the absence (−) or presence (+) of the proteasome inhibitor Bortezomib. Neurons were immunostained for cleaved Casp6 (cC6) and tubulin (inset). Scale bar, 50 μm. Quantification of axon degeneration is shown on the right. (b) Cell bodies of neurons treated as described inawere immunostained for cleaved Casp3 (cC3). Nuclei were labelled with Hoechst. Scale bar, 20 μm. Quantification of cleaved Casp3-positive cell bodies is shown on the right. (c) Cell bodies of neurons treated as described inawere immunostained for cleaved Casp9 (cC9) and nuclei were labelled with Hoechst. Scale bar, 20 μm. Quantification of cleaved Casp9-positive cell bodies is shown on the right. (d) WT and Casp3-deficient neurons were locally deprived with (+) and without (−) Bortezomib and probed for tubulin. NGF-maintained neurons served as controls. Scale bar, 50 μm. Quantification of axon degeneration is shown on the right. All data represent the mean±s.e.m. (n=3). AllP-values were calculated using an unpairedt-test. Figure 5: The proteasome restricts caspase activation to axons during axon-specific degeneration. ( a ) Wild-type (WT) neurons were NGF maintained or locally deprived in the absence (−) or presence (+) of the proteasome inhibitor Bortezomib. Neurons were immunostained for cleaved Casp6 (cC6) and tubulin (inset). Scale bar, 50 μm. Quantification of axon degeneration is shown on the right. ( b ) Cell bodies of neurons treated as described in a were immunostained for cleaved Casp3 (cC3). Nuclei were labelled with Hoechst. Scale bar, 20 μm. Quantification of cleaved Casp3-positive cell bodies is shown on the right. ( c ) Cell bodies of neurons treated as described in a were immunostained for cleaved Casp9 (cC9) and nuclei were labelled with Hoechst. Scale bar, 20 μm. Quantification of cleaved Casp9-positive cell bodies is shown on the right. ( d ) WT and Casp3-deficient neurons were locally deprived with (+) and without (−) Bortezomib and probed for tubulin. NGF-maintained neurons served as controls. Scale bar, 50 μm. Quantification of axon degeneration is shown on the right. All data represent the mean±s.e.m. ( n =3). All P -values were calculated using an unpaired t -test. Full size image Another factor that can restrict caspase activation during axon-specific degeneration is XIAP, which is a potent endogenous inhibitor of caspases in neurons [12] . Owing to the requirement of two critical targets of XIAP (Casp9 and Casp3) for axon degeneration, we predicted that XIAP-deficient neurons may be more vulnerable to caspase-mediated degeneration during local deprivation. Indeed, XIAP-deficient neurons degenerated their axons earlier than wild-type neurons ( Fig. 6a ; Supplementary Fig. S3b ). Also, significantly more Casp3 activation was observed in the cell bodies of locally deprived XIAP-deficient neurons compared with wild-type neurons ( Fig. 6b ). These results show that caspase activation during axon-selective degeneration is spatially restricted by the activities of the proteasome and XIAP. 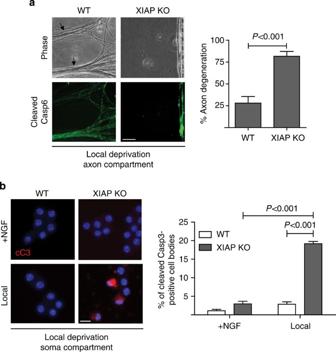Figure 6: XIAP protects the soma from caspase activation during axon-specific degeneration. (a) Wild-type (WT) or XIAP-deficient neurons were locally deprived and probed for cleaved Casp6. Arrows indicate early signs of axonal collapse. Scale bar, 50 μm. Quantification of axon degeneration is shown on the right. (b) WT and XIAP-deficient neurons were NGF-maintained or locally deprived and cell bodies were probed for cleaved Casp3 (cC3). Nuclei were labelled with Hoechst. Scale bar, 20 μm. Quantification of the percentage of cell bodies positively labelled for cleaved Casp3 is shown on the right. All data represent the mean±s.e.m. (n=3). AllP-values were calculated using an unpairedt-test. Figure 6: XIAP protects the soma from caspase activation during axon-specific degeneration. ( a ) Wild-type (WT) or XIAP-deficient neurons were locally deprived and probed for cleaved Casp6. Arrows indicate early signs of axonal collapse. Scale bar, 50 μm. Quantification of axon degeneration is shown on the right. ( b ) WT and XIAP-deficient neurons were NGF-maintained or locally deprived and cell bodies were probed for cleaved Casp3 (cC3). Nuclei were labelled with Hoechst. Scale bar, 20 μm. Quantification of the percentage of cell bodies positively labelled for cleaved Casp3 is shown on the right. All data represent the mean±s.e.m. ( n =3). All P -values were calculated using an unpaired t -test. Full size image Mature neurons inhibit apoptosis but permit axon pruning Our results thus far show that the axon degeneration and apoptosis pathways are distinct but share several key components. One question this raises is whether neurons can shut off apoptosis while maintaining the ability to undergo axon-selective degeneration. Mature neurons provide an excellent model to examine this point because neurons are known to restrict the apoptotic pathway with maturation, in part by turning off the expression of Apaf-1 (ref. 26 ). Specifically, we and others have shown that global NGF deprivation induces apoptosis in young (5 days in vitro , or DIV) but not mature (28 DIV) neurons ( Fig. 7a ) (refs 4 , 5 , 6 , 7 ). 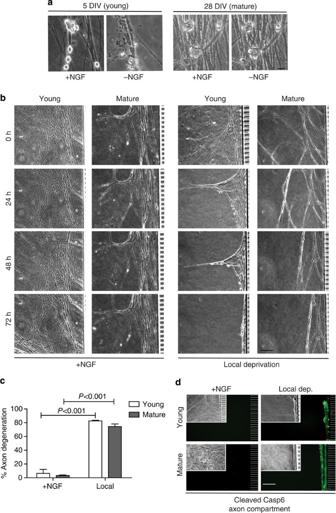Figure 7: Mature neurons inhibit apoptosis during global deprivation but degenerate axons during local deprivation. (a) Young (5 DIV) and mature (28 DIV) sympathetic neurons were either NGF maintained or NGF deprived for 48 h. Scale bar, 20 μm. (b) The same axons of young and mature neurons were imaged every 24 h during local deprivation. NGF-maintained neurons at both ages served as controls. Scale bar, 50 μm. (c) Quantification of axon degeneration for conditions shown inb. Data represent the mean±s.e.m. (n=3). (d) Cleaved Casp6 immunostaining and corresponding phase images (inset) in the axon compartments of conditions shown inb. AllP-values were calculated using an unpairedt-test. Figure 7: Mature neurons inhibit apoptosis during global deprivation but degenerate axons during local deprivation. ( a ) Young (5 DIV) and mature (28 DIV) sympathetic neurons were either NGF maintained or NGF deprived for 48 h. Scale bar, 20 μm. ( b ) The same axons of young and mature neurons were imaged every 24 h during local deprivation. NGF-maintained neurons at both ages served as controls. Scale bar, 50 μm. ( c ) Quantification of axon degeneration for conditions shown in b . Data represent the mean±s.e.m. ( n =3). ( d ) Cleaved Casp6 immunostaining and corresponding phase images (inset) in the axon compartments of conditions shown in b . All P -values were calculated using an unpaired t -test. Full size image To examine whether mature neurons remain permissive for axon-selective degeneration despite shutting down their apoptosis pathway, we subjected young and mature neurons to local NGF deprivation. Our results show that mature neurons are fully capable of activating Casp6 and undergoing axon-selective degeneration as removal of NGF from just the axons triggered axon degeneration ( Fig. 7b–d ). These results are particularly striking as removal of NGF from the entire mature neuron (soma and axons) induces neither apoptosis nor axon degeneration ( Fig. 7a ). Thus, the ability of mature neurons to be permissive or resistant to axon degeneration depends not only on whether NGF is deprived from the axons but also whether it is present or absent in the soma. Taken together, our results have identified key differences in the axon degeneration pathway depending on whether the context is apoptosis or axon-selective pruning ( Fig. 8 ). 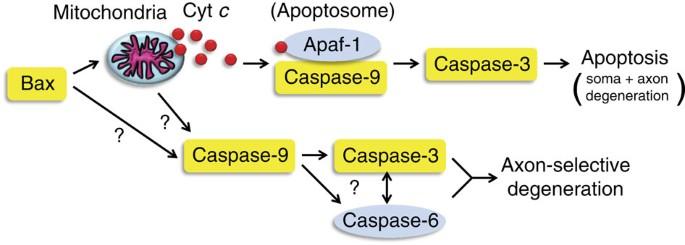Figure 8: Working model of the pathways mediating apoptosis versus axon pruning. Proteins highlighted in yellow have been shown to be required for both apoptosis and axon pruning pathways. Our results indicate that Apaf-1 and Caspase-6 (highlighted in blue) are two points of divergence. Future experiments will be required to determine what role, if any, is played by the mitochondria and cytcrelease in axon-selective degeneration. In addition, how Caspase-9 is able to activate Caspase-6 and Caspase-3 without Apaf-1 remains to be determined. While Caspase-6 and Caspase-3 are both required for axon pruning, their exact order of activation during axon pruning in neurons is still unclear. Figure 8: Working model of the pathways mediating apoptosis versus axon pruning. Proteins highlighted in yellow have been shown to be required for both apoptosis and axon pruning pathways. Our results indicate that Apaf-1 and Caspase-6 (highlighted in blue) are two points of divergence. Future experiments will be required to determine what role, if any, is played by the mitochondria and cyt c release in axon-selective degeneration. In addition, how Caspase-9 is able to activate Caspase-6 and Caspase-3 without Apaf-1 remains to be determined. While Caspase-6 and Caspase-3 are both required for axon pruning, their exact order of activation during axon pruning in neurons is still unclear. Full size image Neurons have the unique capability to activate pathways that cause degeneration of either the entire cell or only the axons [33] . The picture that is emerging is that neurons engage multiple pathways for triggering axon degeneration that is stimuli-specific. Our results now show that even in the context of one stimulus (for example, NGF deprivation), the spatial origin of the stimuli is a key determining factor for activating a specific axon degeneration pathway. We find Casp6 to be activated during axon degeneration but selectively in the context of NGF deprivation. Indeed, axon degeneration after axotomy, termed Wallerian degeneration [34] , and axon degeneration induced by other insults such as microtubule destabilization are likely mediated by an alternate, Casp6-independent mechanism [17] , [20] . The observation that neurons activate a specific pathway for axon degeneration that responds selectively to NGF deprivation is consistent with the relevance of NGF as a physiological factor that regulates sympathetic neuron innervations [35] . Importantly, we find that even in the context of NGF deprivation, Casp6 is essential for axon degeneration only during axon-specific but not whole-cell breakdown. Thus, axon degeneration appears to be critically dependent on Casp6 when the insult is physiologically relevant and spatially localized to axons. Our results also make the critical distinction between axon degeneration that occurs during apoptosis versus axon-selective pruning. While we and others show that Bax, Casp9 and Casp3 are required for axon degeneration [13] , [16] , [17] , [19] , [20] , we report the novel finding that Apaf-1 is not required for this process. These results were unexpected because the major known mechanism for activating Casp9 is via Apaf-1. Incidences of Apaf-1-independent Casp9 activation have been reported in non-neuronal models, yet the mechanism remains unknown [36] , [37] , [38] . Our results showing that mature neurons, which lack Apaf-1 (ref. 26 ), were fully capable of axon degeneration further supports the model of axon-selective pruning as an Apaf-1-independent process. Triggering the complete apoptotic pathway in axons can be especially dangerous for neurons, which are post-mitotic cells that must survive long term. Thus, neurons may utilize a non-apoptosome mechanism of activating Casp9 during axon pruning to tightly restrict the direct activation of Casp3, therefore avoiding the risk of a lethal and widespread apoptotic caspase cascade. Increasing evidence indicates that neurons utilize Bax, Casp9 and Casp3 for synaptic plasticity [39] . We predict that caspase activation under these non-apoptotic conditions may also occur by a pathway that is Apaf-1-independent. Also, while we find cyt c to be released from the mitochondria in degenerating axons, determining whether it is required for Apaf-1-independent Casp9 activation needs further investigation. Experiments that knockdown cyt c are problematic due to the essential function of cyt c in mitochondrial respiration. However, one potential alternative approach would be to introduce neutralizing antibodies to cyt c into axons and assess whether axonal degeneration is prevented. The exact non-apoptosome mechanism by which Casp9 activates the downstream caspases, Casp6 and Casp3, remains unclear. A recent study found Casp3 deficiency to block Casp6 activation, placing Casp6 downstream of Casp3 in this pathway [20] . While we found Casp6 activation to be reduced in Casp3-deficient axons during local deprivation, it was nevertheless detectable ( Fig. 3a ). Importantly, this reduced level of Casp6 activation was incapable of inducing axon degeneration as axonal integrity was maintained in the locally deprived Casp3-deficient neurons. Thus, while Casp3 appears to be needed for the full activation of Casp6 during axon pruning, the exact mechanism of this caspase activation appears more complex than a linear pathway. Our results also identify the proteasome and XIAP as two mechanisms by which neurons limit caspase activity during axon-selective degeneration. Casp6 is a known target of the proteasome [31] , [32] and endogenous XIAP is a potent inhibitor of caspases in neurons [12] . The protective function of XIAP in the cell body during axon-specific degeneration is similar to the mechanism in Drosophila where DIAP (the insect homologue of XIAP) regulates caspase activity during developmental dendritic pruning [40] , [41] . Our results indicate that neurons have evolved multiple mechanisms for restricting axonal caspase activity in order to remodel axons without risking long-term survival. Extensive neuronal apoptosis and axon pruning are both required to establish specific neuronal circuitry during development [3] , [8] . However, whereas the apoptotic pathway becomes highly restricted once neurons are integrated into the nervous system to enable neurons to survive for the lifetime of the organism [4] , [5] , [6] , [7] , the selective pruning of axons is continually required to permit plasticity in the adult nervous system [8] , [9] , [10] . Indeed, we find mature neurons to fully restrict apoptosis yet remain capable of undergoing axon-specific degeneration. Aberrant activation of axon pruning mechanisms in the mature nervous system could contribute to pathological axon degeneration in neurodegenerative disease. While inhibiting caspases could be a potential therapy in these situations, one concern is that chronic administration of caspase inhibitors may also inhibit physiological pruning and synaptic plasticity. Together, our results reveal that neurons are exquisitely capable of discerning the spatial location of NGF signal loss and activating an appropriate response. Neurons appear to utilize essentially the same components for whole cell and axon-selective degeneration yet have evolved distinct mechanisms to allow precise spatial and temporal control over the activation of these pathways. Mice All animal handling and protocols were carried out in accordance with established practices as described in the National Institutes of Health Guide for Care and Use of Laboratory Animals and as approved by the Animal Care and Use Committee of the University of North Carolina. Casp6-deficient mice were obtained from Jackson Labs. Mice deficient for Casp9, Apaf-1 or Casp3 were dissected at E16.5 due to the embryonic lethality often associated with these gene deficiencies at later ages. All knockout mice were on a C57BL/6 background, and wild-type littermates served as controls for all experiments. Primary sympathetic neuronal cultures Primary sympathetic neurons were cultured as previously described [12] . Briefly, sympathetic neurons were dissected from the superior cervical ganglia of postnatal day (P)0-1 CD1 mice. Cells were plated on collagen-coated dishes at a density of 10,000 cells per well or in microfluidic chambers (see section below) and maintained for 5 days in vitro (DIV) in NGF-containing medium (AM50). For NGF deprivation, cultures were rinsed three times with medium lacking NGF (AM0) and then maintained in NGF-deficient media containing a neutralizing antibody to NGF. Some neuronal cultures were treated with various compounds in the presence of NGF: 20 μM etoposide; 2.5 μM tunicamycin; 1 μM vinblastine. All reagents were obtained from Sigma unless otherwise indicated. All experiments were performed in triplicate. Fabrication and use of microfluidic devices Standard photolithography was used to fabricate channel array devices for axon growth. Negative photoresist (KMPR 1010, MicroChem Corp., Newton, MA) was used to pattern arrays of 10-μm wide, 3-μm deep grooves spaced 40 μm apart onto a standard silicon wafer (Silicon Quest International). The bare silicon around the pattern was etched ~3-μm deep using deep reactive ion etching (Alcatel AMS 100 Deep Reactive Ion Etcher) with a low-roughness Bosch process. The photoresist was then stripped using 2,800 W oxygen plasma. The features for the large side compartments (750-μm long, 100-μm deep, 1.0-mm wide on each side) at either end of the central grooves were fabricated onto the wafer using negative photoresist (SU8-100, MicroChem Corp.) and standard photolithography using the manufacturer’s recommended procedure. Sylgard 184 (Dow Corning) was prepared according to the manufacturer’s recommended procedure and poured into the mould form. After curing at 65 °C overnight, individual polydimethylsiloxane (PDMS) chambers were cut out, sterilized in 70% EtOH and placed upon glass coverslips coated with 40 μg ml −1 poly- D -lysine (BD Biosciences) and 0.1 μg ml −1 mouse laminin (Invitrogen). Culture and treatment of primary neurons Neurons were plated in microfluidic chambers as described previously [24] and maintained in AM50 until 5 DIV (or 28 DIV for mature experiments). To achieve global deprivation of NGF, both compartments were carefully rinsed three times with AM0 and then maintained in AM0 containing NGF-neutralizing antibodies. For local deprivation only the axon compartment was rinsed and deprived of NGF, whereas the soma compartment was maintained in AM50. Chambers containing AM50 in both compartments served as controls. A 30-μl volume differential was established between the two compartments at the start of treatment and reset every 12–20 h to maintain fluidic isolation [24] . Where indicated, 25 μM zIETD-FMK (Casp8-specific inhibitor, SM Biochemicals) or 25 μM QVD (quinolyl-Val-Asp-OPh, pancaspase inhibitor, SM Biochemicals) was added at time of treatment. Also, 10 μM Bortezomib was added 8–10 h into treatment to preclude any toxic effects resulting from longer proteasome inhibition. Quantification The length of intact axons was measured both before and after treatment. The left edge of the chamber’s microgrooves (where axons first enter the axon compartment) served as the starting point of measurement. Distinct markers were imprinted on the microgrooves during the chamber design and fabrication process to allow identification of the same axons and chamber regions over time. It is important to note that fragmented axons do not remain adhered to the glass coverslip; very slow media flow within the chamber compartment, coupled with the absence of a ‘sticky’ matrix such as collagen or methylcellulose, removes away the degenerated axon pieces. The microfluidic chamber system permits very clear detection of maintained, adherent and intact axons versus degenerating and non-adherent axons (see phase time course images in Figs 3d and 7b ). Therefore, we compared the length of intact axons both before and after treatment to determine the percentage of each measured axon that was maintained and, inversely, the percentage of each measured axon that was lost as a result of treatment-induced degeneration. Immunofluorescence Immunofluorescence staining was carried out as previously described [12] . Briefly, cultures were gently rinsed in phosphate-buffered saline and fixed in fresh 4% paraformaldehyde at room temperature for 20 min. Cultures were rinsed three times with Tris-buffered saline and exposed to blocking solution (Tris-buffered saline containing 5% donkey serum and 0.3% Triton X-100) for 1 h at room temperature. Following blocking, cells were treated with primary and secondary antibodies using standard methods and nuclei were labelled with the nuclear dye bisbenzimide (Hoechst 33258 at 1 μg ml −1 , Invitrogen). The same steps were carried out in microfluidic chambers by gradually adding solutions to the reservoirs to ensure proper flow into the soma and axon compartments. For experiments involving knockout neurons, cells were fixed when neurons from wild-type littermates showed extensive axon degeneration following treatment. The following primary antibodies were used for immunostaining: cleaved Caspase-6 (Santa Cruz, 1:200), cleaved Caspase-3 (Cell Signaling, 1:400), cleaved Caspase-9 (Cell Signaling, 1:400), cytochrome c (Molecular Probes, 1:400), Tom20 (Santa Cruz, 1:400) and tubulin (1:400). Tyramide signal amplification (Molecular Probes) was used according to manufacturer’s instructions to visualize cleaved Casp3 in axons and cleaved Casp9. Image acquisition and processing Images were acquired by an ORCA-ER digital B/W CCD camera (Hamamatsu) mounted on a DMIRE2 inverted fluorescence microscope (Leica) using Metamorph version 7.6 software (Molecular Devices). Statistical analysis All P -values were calculated using an unpaired t -test. How to cite this article: Cusack, C. L. et al . Distinct pathways mediate axon degeneration during apoptosis and axon-specific pruning. Nat. Commun. 4:1876 doi: 10.1038/ncomms2910 (2013).